A general11C-labeling approach enabled by fluoride-mediated desilylation of organosilanes Carbon-11 ( 11 C) is one of the most ideal positron emitters for labeling bioactive molecules for molecular imaging studies. The lack of convenient and fast incorporation methods to introduce 11 C into organic molecules often hampers the use of this radioisotope. Here, a fluoride-mediated desilylation (FMDS) 11 C-labeling approach is reported. This method relies on thermodynamically favored Si-F bond formation to generate a carbanion, therefore enabling the highly efficient and speedy incorporation of [ 11 C]CO 2 and [ 11 C]CH 3 I into molecules with diversified structures. It provides facile and rapid access to 11 C-labeled compounds with carbon-11 attached at various hybridized carbons as well as oxygen, sulfur and nitrogen atoms with broad functional group tolerance. The exemplified syntheses of several biologically and clinically important radiotracers illustrates the potentials of this methodology. Positron emission tomography (PET) is a clinical and research imaging modality for the non-invasive investigation of biochemical and molecular events in living organisms using radioactive positron emitting tracers. In the past two decades, the application of PET to the study of various diseases (oncological, neurological and cardiovascular) has positioned this modality as one of the most powerful translational imaging tools available. Among several short-lived positron-emitting radionuclides used in PET imaging, carbon-11 ( 11 C, t 1/2 = 20.4 min, E β+ = 1.98 MeV) stands out as unique [1] , [2] , [3] . The ubiquitous presence of carbon in organic molecules makes 11 C an attractive and important positron-emitting radionuclide for labeling a vast array of molecules of biological interest. Importantly, 11 C-labeled molecules possess the same chemical and biological properties as the non-radioactive 12 C-molecule of interest; thus making 11 C extraordinarily useful for the exploration of molecules with well-characterized biological and pharmacological properties (i.e., metabolism, drug pharmacokinetics, receptor binding affinity, enzyme substrate affinity, etc.). In addition, the short half-life of 11 C enables the possibility of performing multiple imaging studies in the same subject on a single day, which is especially beneficial for clinical researches. This unique utility of 11 C demands that there be rapid and robust approaches available to incorporate 11 C into various organic molecules in an efficient manner. Carbon-11 labeled PET tracer syntheses generally start with the cyclotron production of [ 11 C]CO 2 or [ 11 C]CH 4 , which are produced by the proton bombardment of N 2 gas (doped with O 2 or H 2 ) using the 14 N(p,α) 11 C nuclear reaction. The most commonly produced radioactive intermediate [ 11 C]CO 2 , can be either used directly as a primary radiosynthon or be rapidly converted to more reactive secondary radiosynthons ([ 11 C]CH 3 I, [ 11 C]CH 3 OTf, [ 11 C]HCN, [ 11 C]HCHO, [ 11 C]CO, [ 11 C]COCl 2 , etc. ), enabling a variety of radiosynthetic strategies. After postreaction purification, typically using chromatographic and/or solid phase extraction (SPE) techniques, the desired 11 C-labeled tracer is isolated and formulated for use in preclinical or clinical studies. The main challenge for a successful synthesis of 11 C-labeled PET tracers is a rapid, robust, and practical radiolabeling method that yields a desired tracer dose of pharmaceutically acceptable quality, i.e. high radiochemical & chemical purity, and typically high specific activity ( A s ) or molar activity ( A m ). In addition, such a method should be easily adapted for automation to minimize radiation exposure to the operator, and the labeling precursors should be either commercially available or readily synthesized [1] , [2] , [3] . [ 11 C]CO 2 has been directly used for PET tracer synthesis for decades. It is now routinely produced for the synthesis of carbon-11 labeled fatty acids such as [ 11 C]acetic acid and [ 11 C]palmitic acid via the Grignard reaction in many PET facilities worldwide. However, because of its inertness, radiolabeling reactions using [ 11 C]CO 2 generally require the use of strong organometallic reagents, such as Grignard and organolithium reagents, which are sensitive to moisture and atmospheric 12 CO 2 and less tolerant to the presence of various functional groups. These drawbacks impede the broader application of [ 11 C]CO 2 for synthesizing highly functionalized molecules. To expand the utility of [ 11 C]CO 2 for the synthesis of PET tracers with diverse structures, including multiple functional groups, researchers have recently reported on both the incorporation of [ 11 C]CO 2 into molecules under milder conditions, and the introduction of 11 C to specific positions that are not easily achieved using other secondary radiosynthons [4] , [5] , [6] , [7] , [8] , [9] , [10] . Despite such developments, the method of directly incorporating [ 11 C]CO 2 for synthesis of 11 C-labeled radiotracers remains sorely lacking in the field of PET chemistry. Hence, there is a heretofore unmet need to develop radiolabeling methodologies that can directly and promptly introduce [ 11 C]CO 2 to molecules with diverse structure and/or containing multiple functional groups under mild reaction conditions. Herein, we report our recent development of a fluoride-mediated desilylation (FMDS) 11 C-labeling approach derived from a fluoride desilylation promoted nucleophilic reaction [11] . Carbon-11 labeled carboxylic acids containing various functional groups with 11 C attached at different hybridized carbons (sp, sp 2 , and sp 3 ) are synthesized by in situ generation of various nucleophiles via fluoride agents and organosilanes, followed by a quick 11 C-carboxylation reaction. Moreover, this method is also readily extended to label organic molecules with [ 11 C]CH 3 I as the radiolabeling synthon. Synthesis of [ 11 C]acetoacetic acid via FMDS 11 C-carboxylation To support the PET imaging study of the metabolic process of ketone bodies in brain tumors, we recently developed a production method for [ 11 C]acetoacetic acid ( [ 11 C]3 ) following a literature method [12] , [13] , in which isopropenyl acetate, 1 , was first reacted with methyl lithium to form lithium enolate, 2 . Next, the enolate, 2 , was used for reacting with [ 11 C]CO 2 to form the desired product [ 11 C]3 (Fig. 1a ). One of the difficulties encountered in the production process was that the chemical impurities were occasionally detected in the final product and proved difficult to remove using standard purification methods. To assure robust production of a high quality [ 11 C]3 tracer, we sought to develop a different approach to [ 11 C]CO 2 incorporation under milder conditions, such conditions would avoid the use of a harsh organometallic reagent, which not only generated the desired enolate but also caused some side reaction(s). After an extensive literature search, we found that a fluoride ion desilylation enolate generation method reported by Noyori in 1983 could be amenable for this purpose [14] . Fig. 1: Methods for synthesizing [ 11 C]3. Two cGMP-compliant synthesis methods for preparing [ 11 C ] 3. a organolithium method; c FMDS 11 C-carboxylation method, and mechanistic explanation of formation of [ 11 C ] 3 via FMDS 11 C-carboxylation approach ( b ). Full size image The exploration of a FMDS 11 C-carboxylation strategy for synthesis of [ 11 C]3 began by using (isopropenyloxy)trimethylsilane, 4 , as the organosilane reagent and tris(dimethylamino)sulfonium difluorotrimethylsilicate (TASF) as the fluoride ion source [14] , [15] . Binary solvent systems (tetrahydrofuran (THF) and dichloromethane (DCM)) were employed for the reaction due to the low solubility of TASF in THF [16] . The initial experiment provided us [ 11 C]3 with a 5% radiochemical yield (RCY, based on HPLC analysis of the crude product). The formation of [ 11 C]3 via FMDS 11 C-carboxylation approach could be understood from the mechanistic scheme in Fig. 1b . The driving force of the enolate anion formation under such mild conditions comes from the strength of the silicon-fluorine bond (139 kcal/mol), which makes enolate generation via fluoride-mediated desilylation as a thermodynamically favored process [14] . After several preliminary experiments, the RCY (based on HPLC analysis of the crude product) of [ 11 C]3 quickly improved to over 50%. However, purification with either ion-exchange or semi-prep HPLC methods failed to provide a product with acceptable chemical purity. This was due to the large amount of TASF reagent and water incompatible solvent DCM used for reactions. At this stage, cesium fluoride (CsF) was tested as a replacement for TASF to overcome these problems [17] , [18] . The modification of experimental conditions (such as using THF and dimethylformamide (DMF) (3/1, V/V) binary solvents, trapping [ 11 C]CO 2 at low temperature, pre-drying the CsF reagent using azeotropic evaporation, adjusting the quantity of the ion exchange resin as well as introducing an Al–N cartridge at the end of the purification process for removal of extra fluoride ion) dramatically improved the overall reaction yield and the chemical purity of the final product. An optimized synthetic protocol (Fig. 1c ) was developed that was suitable for production under cGMP compliant conditions. The product [ 11 C]3 was synthesized with high radiochemical purity (RCP, 95.9 ± 1.5%) and high RCY (57.4 ± 8.1%, n = 3; decay corrected, DC), in a similar time frame (from end of [ 11 C]CO 2 collection to end of product collection, 28.7 ± 5.5 min) compared with the results of the organolithium reagent based method (RCP, 97.1 ± 1.1%; RCY, 24.4 ± 2.0%; 24.0 ± 2.6 min, n = 3). It is noticeable that both production processes developed by us needed longer production time comparing with the automated production reported by Sébastien Tremblay, et al in 2007 (RCY, 34 ± 5%; 18 min, n = 20) [12] . The development of automated synthesis process in the future, hopefully, could help us to shorten the whole production time. An important feature of this updated method is that both reagents used (enol silyl ether, 4 , and CsF), unlike organometallic reagents, are not sensitive to atmospheric 12 CO 2 . In addition, CsF can be easily dried using an azeotropic distillation method which means greater ease in handling of reagents and less stringent operating conditions for production of this clinically useful radiotracer. Exploration of synthesis of 11 C-carboxylates and derivatives The success in developing an updated method for synthesizing [ 11 C]3 triggered our interest in exploring carbon nucleophiles, generated in situ via FMDS approach, for 11 C-carboxylation. Although FMDS method had been used to generate a variety of nucleophiles in many organic reactions (such as alkylation, allylation, alkynylation, arylation, vinylation, and cyanation), and had been broadly used to synthesize complex molecules [11] , there are only a handful of reports of directly using organosilanes for carboxylation reaction without involving any transition metal catalysts [19] , [20] , [21] , [22] , [23] , [24] , [25] , [26] , [27] , [28] , [29] . While organometallic reagent catalyzed carboxylation has already drawn extensive attention to radiochemistry research [30] , [31] , [32] , to the best of our knowledge, we have not found any reports of the use of the FMDS methodology for direct 11 C-carboxylation. It is comprehensible that the high cost and necessity of stoichiometric amounts of organosilane reagents made this method less attractive in synthetic organic chemistry research when compared to other organometallic reagent catalyzed carboxylation methodologies [33] , [34] . For 11 C-labeled radiotracer production, however, the primary costs come from cyclotron bombardment for generation of [ 11 C]CO 2 , highly complex equipment-dependent automated synthesis, and elaborate quality control processes. The quantities of chemicals required for 11 C-labeling reactions are at the micromole and milliliter level, hence the cost of reagents is in a minor consideration. Based upon these prerequisites, adopting a FMDS strategy for 11 C-carboxylation provides many potential advantages, such as: (1) The simplicity of the whole reaction system, since only four reagents (organosilane, fluoride source, solvent, [ 11 C]CO 2 ) are involved in the labeling reactions and there is no organometallic catalyst, ligand(s), base, etc. needed; (2) Less precaution is needed for preparation compared with organometallic reagent based 11 C-carboxylation methods since most organosilanes and fluoride source (such as CsF) are not sensitive to atmospheric 12 CO 2 . This difference implies another advantage, i.e. the 11 C-labeled PET tracers with high molar activity could be obtained under less stringent conditions; (3) The mildness of the FMDS 11 C-labeling strategy could help us to synthesize 11 C-carboxylic acids and their derivatives attached to compounds with diversified functional groups thereby dramatically broadening the scope of 11 C-labeling via direct use of [ 11 C]CO 2 as a radiosynthon. We first explored 11 C-carboxylation using alkynyltrimethylsilanes, 6 , and CsF for sp-hybridized carbanion generation [35] . After preliminary tests, it was found that a combination of THF and dimethyl sulfoxide (DMSO) worked better for these 11 C-carboxylation reactions, which stoichiometric reagent ([ 11 C]CO 2 and [ 12 C]CO 2 together) at nano- or subnano-moles level, than DMSO alone (Fig. 2 ) [27] . The selected reaction conditions not only trapped [ 11 C]CO 2 efficiently (usually >90% [ 11 C]CO 2 radioactivity was retained in the reaction mixture), but also transferred it into 3-substituted propiolic-[1- 11 C]acid upon heating the reaction mixture at 40 °C for 5 min with excellent radiochemical yield (RCY, [ 11 C]7a-b, e-f , ranging from 72.4 to 98.5%; all radiochemical yields displayed for the rest of work were determined by multiplying the radiochemical purity as determined by HPLC times isolated radioactivity divided by the starting [ 11 C]CO 2 (decay corrected), unless stated otherwise) despite the difference in functional groups (either electron withdrawing or donating) and their positions in the phenyl ring ( ortho , para , or meta ). The replacement of DMSO with DMF was less impactful for the 11 C-carboxylation (3-(4-bromophenyl)propiolic-[1- 11 C]acid, [ 11 C]7c , yield = 66.5 ± 11.8%). In addition, the 11 C-carboxylation conditions were also adaptable with naphthalenyl ( 6g ), 3-thienyl ( 6h ), methyl, and ethyl esters ( 6i and 6k ), and chloropropyl groups ( 6j ) attached ethynyltrimethylsilanes and all reagents provided the corresponding 3-substituted propiolic-[1- 11 C]acids, [ 11 C]7g-k , with excellent yields as well. Decreasing the amount and concentration of precursor ( 6k , 0.05 mmol and 0.167 M vs 6i , 0.25 mmol and 0.33 M) only slightly decreased the incorporation of [ 11 C]CO 2 into the desired 3-substituted propiolic-[1- 11 C]acid (yields of [ 11 C]7i and [ 11 C]7k , 95.8 ± 4.0% vs 87.7 ± 7.5%). Fig. 2: FMDS 11 C-carboxylation with sp-hybridized carbon attached trimethylsilanes. Unless otherwise indicated, the reported values are radiochemical yields (RCY, n = 3) of determined by radio-HPLC analysis of the crude product and the product identities were determined by co-injection with corresponding carbon-12 standards. a THF (0.5 mL) + DMF (0.25 mL) were used; b Reaction was maintained at r.t., 2 min; c DMSO was used as solvent; d Precursor (0.029 mmol, 5 mg) and DMF (0.3 mL) were used for reactions. Full size image To further demonstrate the versatility of this 11 C-carboxylation method, we explored the amenability of a quick conversion of 11 C-carboxylic acids into their ester and amide derivatives (Fig. 2 ) [5] . The desired product, 3-pyridyl attached methyl [1- 11 C]propiolate, [ 11 C]9 , was formed with a 28.0 ± 2.6% yield without any optimization of reaction conditions by the 11 C-carboxylation reaction of alkynyltrimethylsilanes, 7l , followed with the methyl esterification by adding methyl iodide (0.75 mmol) to the same reaction vial and heating at 40 °C for 5 min. The transformation of 11 C-carboxylic acid into carboxamide was also exemplified by smoothly converting [ 11 C]carboxylic acid, [ 11 C]7f , to its benzylamide derivative, [ 11 C]9 [5] . As an intermediate, [ 11 C]7f was first purified using solid phase extraction (SPE) technique with a C18 plus cartridge. The radioactivity was then eluted from the cartridge using THF into a second reaction vial, and reacted with N -hydroxysuccinimide (HOSu) and dicyclohexylcarbodiimide (DCC) at 60 °C for 5 min. The desired benzylamide derivative, [ 11 C]9 , was formed by adding benzylamine (1.0 mmol) and heating the reaction mixture at 60 °C for 5 min with an overall yield of 20.6%. Upon successful addition of the 11 C-carboxylate moiety at sp-hybridized alkynyl carbons, we immediately turned our focus to different organosilane substrates, specifically trimethylsilyl (TMS) groups attached at the sp 2 -hybridized carbon, for synthesizing 11 C-carboxylic acids using FMDS 11 C-carboxylation approach (Fig. 3 ). Unlike the synthesis of various 11 C-propiolates, in which the reaction parameters required minor variation, the reaction temperature for the synthesis of different aryl/heteroaryl 11 C-carboxylic acids, [ 11 C]11 , had to be modified significantly. Acetophenone enol trimethylsilyl ether, 10a , similar to silyl enol ether 4 , displayed high reactivity and the β -carbonyl [ 11 C]carboxylic acid, [ 11 C]11a , was obtained with a 71.3 ± 15.1% yield under similar reaction conditions as propiolic-[1- 11 C]acids, with only a change of solvent to DMF. The di- and tri-halide substituted trimethylsilylbenzene, 10b and 10c , displayed high propensity to convert to the corresponding [ 11 C]benzoic acids, [ 11 C]11b and [ 11 C]11c with excellent conversion yields. The substrate reactivity dropped significantly when the halide groups were moved from ortho- to meta- positions and when one fluorine was changed to bromine ( [ 11 C]11c vs [ 11 C]11d , 60 °C, 5 min, 84.6 ± 4.3% vs 170 °C, 8 min, 18.8 ± 1.8%) [24] . The removal of one bromide group from meta- position further decreased the reactivity of the substrate and the reaction temperature had to be increased to 180 °C to maintain comparable reaction yields ( [ 11 C]11e , 19.4 ± 7.1%). The change of the bromide group from meta- to para- position further reduced reaction yields and only 11.1 ± 1.8% of the desired 4-bromo-[1- 11 C]benzoic acid, [ 11 C]11f , was obtained under the same reaction conditions. Fig. 3: FMDS 11 C-carboxylation with sp 2 -hybridized carbon attached trimethylsilanes. a Solvent DMF (0.25 mL) + THF (0.5 mL), precursor is sp 2 -hybridized carbon attached silyl enol ether; b Precursors are highly moisture sensitive; c There was no detected product at 150 and 160 °C; d Precursor 10 mg (0.05 mmol) in DMF (0.3 mL) ( n = 4 for RCC); e tert -Butyldimethylsilyl attached 1-methylimidazole was used as precursor; there was no product detected at 120 °C, 8 min for all reactions. Full size image When trimethylsilylbenzene, 10g , was tested, only 1.4% of desired [ 11 C]benzoic acid, [ 11 C]11g , was observed at extreme conditions (200 °C, 8 min) and no product was detected at lower reaction temperature (150 and 160 °C). The other indolent substrate, (1-naphthyl)trimethylsilane, 10h , showed slightly better reactivity under the same conditions and [ 11 C]11h was obtained with a 5 ± 2.6% yield at lower reactant concentration (0.167 M vs 0.33 M). A similar trend in reactivity was found when pyridyltrimethylsilanes were tested as substrates for 11 C-carboxylation (Fig. 3 ). With the more electron-withdrawing group, fluoro, attached at the ortho- position, the substrate 10i clearly showed higher reactivity (80 °C, 8 min, 20.3 ± 6.0% [ 11 C]11i ) than substrate 10j , which has a less electron negative chloride atom substituted at meta- position of the TMS group (160 °C, 8 min, 22.8 ± 2.0% [ 11 C]11j ). Without the chlorine substitution, 2-trimethylsilylpyridine, 10k , clearly showed weaker reactivity and the product [ 11 C]11k was obtained in lower yields under the same reaction conditions as [ 11 C]11j (160 °C, 8 min, 13.2 ± 2.3%). The other two heteroaryl trimethylsilanes also presented dramatically different reactivity: 2-trimethylsilylbenzothioazole, 10l , displayed a high propensity to form [ 11 C]11l (r.t., 2 min, 74.9 ± 6.2%). While 2-( tert -butyldimethylsilyl)-1-methyl-1 H -imidazole, 10m , exhibited low reactivity with only a 6.5% of the desired [ 11 C]11m even when the reaction mixture was heated to 200 °C for 8 min (only 1.3% [ 11 C]11m was detected with reaction mixture was heated to 160 °C for 8 min). Following the exploratory synthesis of various aryl and heteroaryl 11 C-carboxylic acids, we further extended our investigation to employ FMDS strategy for 11 C-carboxylation using organosilanes with the TMS group attached at the sp 3 -hybridized carbon (Fig. 4 ). Three benzylsilanes showed similar reactivity with or without bromine substituted in the aromatic ring ( 12a and 12b vs 12c ) and these reactions (120–140 °C, 5–8 min) gave the desired [ 11 C]phenyl acetic acids ( [ 11 C]13a-c ) with good yields (54–72%) [28] . Remarkably, two other benzyltrimethylsilane type substrates, (9-trimethylsilyl)fluorine 12d , and bis(1 H -inden-1-yl)dimethylsilane 12e , gave corresponding 11 C-carboxylic acids, [ 11 C]13d - e , with excellent yields even at ambient temperature. A large variation in RCY was seen for methyltrimethylsilanes bearing a variety of substitutions ( 12f-k , Fig. 4 ). Trifluoromethyl trimethylsilane 12f displayed extremely high reactivity and 11 C-carboxylation had to be performed using extreme conditions, i.e., the collection of [ 11 C]CO 2 was processed at −78 °C using THF as the solvent. After [ 11 C]CO 2 trapping, the reaction vessel was maintained at room temperature (r.t.) for 2 min to afford over 90% conversion of [ 11 C]CO 2 to the desired [ 11 C]trifluoroacetic acid, [ 11 C]13f . The extended reaction time (from 2 to 5 min) at r.t. was detrimental to the reaction with a reduced yield of 19%. When dichloromethyl trimethylsilane, 12g , was tested, both the collection of [ 11 C]CO 2 and the reaction were maintained at r.t. and the reaction solvent was switched to a dual solvent system (THF/DMF, 2/1, v/v) to afford [ 11 C]dichloroacetic acid, [ 11 C]13g , with a yield of 39.2 ± 10.7% . The substrate Ethyl 3-(trimethylsilyl)acetate, 12h , needed to be maintained at 40 °C for 5 min to provide monoethyl [1- 11 C]malonate, [ 11 C]13h , with an excellent yield (95.5 ± 0.7%). Interestingly, phenylsulfone and phenylthio substituted methyl trimethylsilanes, 12i and 12j , showed quite different reactivity toward 11 C-carboxylation. The former gave desired product, [ 11 C]13i , with a 86.6 ± 21.4% yield at 60 °C for 5 min. The latter, however, displayed moderate reactivity and provided desired phenylthio substituted [1- 11 C]acetic acid, [ 11 C]13j , with only a 18.8 ± 2.7% yield even when heated at 100 °C for 5 min. It was found that the allyltrimethylsilane derivative, 12k , was less reactive, as the reaction mixture had to be heated to 160 °C for 8 min to produce the corresponding 11 C-carboxylic acid, [ 11 C]13k , with a 19.3 ± 1.8% yield. Fig. 4: FMDS 11 C-carboxylation with sp 3 -hybridized carbon attached trimethylsilanes. a Precursor (0.05 mmol, 12 mg), DMF (0.3 mL); b Reaction vial was maintained at r.t. for 2 min after [ 11 C]CO 2 collection was done at −78 °C, THF as solvent; c Solvent DMF (0.25 mL) + THF (0.5 mL); d Precursor is highly moisture sensitive; e RCY based on n = 4. Full size image The different reactivity of sp-, sp 2 -, and sp 3 -carbon attached organosilanes used in FMDS 11 C-carboxylation reactions can be explained by the p K a value of the conjugate acid of the fluoride-desilylation generated anionic nucleophile [11] . The carbanions generated by FMDS process can be assigned to three groups based upon the p K a values of their conjugate acids: Group 1 (p K a ~20–35) usually form stabilized anions and display high reactivity. Trimethylsilanes ( 4 , 6 , 10a-c , 10l , 12d-i ) all belong to this category. Group 2 (p K a ~35–45) includes carbanions attaching one weakly anion stabilizing group such as allyl, benzyl, and heterocyclic benzyl analogs, and phenylthiomethyl. Aryl groups bearing one or more electron-withdrawing substituents formed carbanions also can be included in Group 2. Trimethylsilane substrates ( 10d-f , 10i-k , 12a-c , and 12j-k ) could be categorized in this group. Last, group 3 contains very weakly stabilized anions (p K a values of their conjugate acids is usually >45). The examples in our study, such as 10g-h and 10m , can be assigned to this category and usually gave minimal (<10% RCY or non-detectable) desired 11 C-carboxylic acids. Extension of FMDS 11 C-labeling approach for 11 C-methylation Bolstered by the success of using FMDS 11 C-carboxylation strategy to synthesize various 11 C-carboxylic acids and their derivatives, we next attempted the translation of this radiolabeling approach for 11 C-methylation. Since methyl iodide (CH 3 I) and methyl triflate (CH 3 OTf) are much better electrophiles compared with the chemically inert CO 2 , we assumed that FMDS 11 C-carboxylation approach should be easily adaptable for 11 C-methylation and the following results supported our speculation. We started exploration of 11 C-methylation using FMDS approach, again, from the protocol reported by Noyori in 1983 [14] . 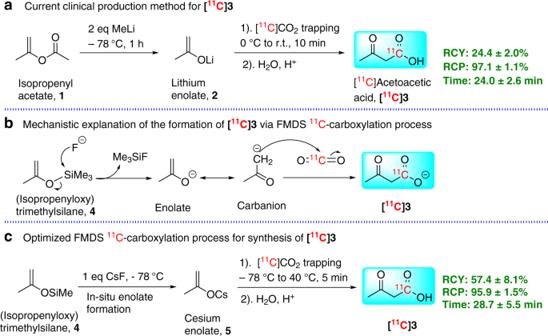Fig. 1: Methods for synthesizing [11C]3. Two cGMP-compliant synthesis methods for preparing [11C]3.aorganolithium method;cFMDS11C-carboxylation method, and mechanistic explanation of formation of [11C]3via FMDS11C-carboxylation approach (b). After screening various experimental conditions (Table 1 ), it was found that the combination of [ 11 C]CH 3 I/CsF/DMF (Table 1 , entry 4) was the optimal choice compared with the more reactive [ 11 C] CH 3 OTf (Table 1 , entry 3) or the more labile fluoride source TASF (Table 1 , entry 1 and 2) [36] . The silyl enol ether, 4 , converted to the desired [4- 11 C]butanone, [ 11 C]14 , with a 43.7 ± 16.4% yield while maintaining the reaction at r.t. for 2 min after the collection of [ 11 C]CH 3 I to the reaction vial (Table 1 , entry 4). Table 1 FMDS 11 C-methylation reaction conditions screening. Full size table With the initial CsF/DMF/[ 11 C]CH 3 I conditions defined, we next evaluated the scope of FMDS 11 C-methylation using a variety of organosilane reagents (Fig. 5 ). All phenoxysilane substrates that were tested gave good to excellent 11 C-methylation yields under mild reaction conditions despite the variation of electron -donating ( 15d-e ), -neutral ( 15a ) or -withdrawing ( 15b , 15b′, 15c , 15f-g ) groups attached at the phenyl ring. The change of tert -butyldimethylsilyl (TBDMS) to triisopropylsilyl (TIPS) ( 15b vs 15b′ ) had minimal impact upon the labeling yields (81.9 ± 1.2% [ 11 C]16b vs 85.7 ± 8.4% [ 11 C]16b ). Even the precursor, 15h , with a phenyl ring that possessed three functional groups afforded excellent reaction yields (81.8 ± 2.7% [ 11 C]16h ). The naphthyl group containing compound tert -butyldimethyl(naphthalen-2-yloxy)silane, 15i , was labile under the reaction conditions. The reactions formed large amount of radioactive by-products even with reactions at r.t. for 5 min and only gave a moderate yield (42.9 ± 13.8% [ 11 C]16i ). The trimethyl(phenylthio)silane, 15j , on the contrary, provided excellent yields (91.3 ± 6.2% [ 11 C]16j ) under the same reaction conditions. Benzyloxytrimethylsilane, 15k , displayed moderate reactivity and the radiolabeling yield only reached 32.7 ± 5.5% ( [ 11 C]16k ) when the reaction mixture was heated at 100 °C for 5 min. Both N -trimethylsilyl substituted substrates gave excellent labeling yields (92.4 ± 2.0% [ 11 C]16l and 93.4 ± 3.1% [ 11 C]16m ) despite quite different reaction conditions (80 °C vs r.t.). The substrate 15n (which is the same as 10m ) displayed excellent reactivity and labeling reactions were performed at r.t. for 5 min to afford 2-(methyl- 11 C)benzo[d]thiazole [ 11 C]16n with a 50.1 ± 8.8% yield. Using the semi-prep HPLC for purification, [3- 11 C]ibuprofen, [ 11 C]16o , was obtained with a 26.6 ± 0.6% yield (based upon the product separated from semi-prep HPLC) from a triethylsilyl (TES) group attached compound 15o after 11 C-methylation at 40 °C for 5 min and saponification by 4 M NaOH. Similar to the synthesis process of [4- 11 C]butanone [ 11 C]14 , Acetophenone enol trimethylsilyl ether, 15p (same as 10a ), was employed as the precursor and TASF as the fluoride reagent, the desired product [3- 11 C]propiophenone, [ 11 C]16p , was synthesized with a 68.2 ± 8.9% yield (based upon the product separated from semi-prep HPLC). Fig. 5: FMDS 11 C-methylation. a tert -Butyldimethylsilyl (TBDMS) group attached compounds as labeling precursors; b Triisopropylsilyl (TIPS) group attached compound as labeling precursor. c Triethylsilyl (TES) group attached ethyl ester as labeling precursor; [ 11 C]CH 3 I was collected at r.t., 3 min, then 40 °C, 2 min; Next saponification: 4 M NaOH, 120 °C, 5 min; products were purified by semi-prep HPLC. d TASF was used as fluoride source, THF (0.5 mL)/DCM (0.25 mL) was used as solvent, [ 11 C]CH 3 I was collected at −40 °C, 3 min, reaction mixture was left at r.t., 2 min, products were purified by semi-prep HPLC; starting radioactivity of [ 11 C]CH 3 I: 7.3 ± 2.67 GBq; total synthesis time: 37.7 ± 1.2 min; radiochemical purity (RCP) > 99% and A m : 29.7 ± 10.9 GBq/µmol (end of bombardment, EOB). Full size image The significance of our FMDS 11 C-labeling method was not only demonstrated by the successful synthesis of thirty seven different 11 C-carboxylic acids, but also exemplified by the in situ quick and smooth conversion of the 11 C-carboxylic acids to their methyl ester and benzylamide derivatives. Additionally, we have readily extended this method to the 11 C-methylation process. The robustness of FMDS 11 C-methylation approach was illustrated by fast and facile synthesis of seventeen different 11 C-methylated compounds with diversified structures by selectively attaching [ 11 C]CH 3 - group to the specific position (oxygen, sulfur, nitrogen and carbon atoms) of these molecules. Exploratory synthesis of three radiotracers As a final demonstration of the strength of FMDS 11 C-labeling method and its feasibility for practical radiotracer production, in addition to the aforementioned cGMP-compliant production of [ 11 C]AcAc ( [ 11 C]3 ), we further explored the practical synthesis of three 11 C-labeled organic molecules, ([ 11 C]raclopride [ 11 C]18 , [ 11 C]succinic acid [ 11 C]19 , and [ 11 C]dichloroacetic acid [ 11 C]13g ), which are of biological and clinical interest but synthetically challenging molecules. To facilitate the regular production and the purification process of these tracers, a lower amount of organosilane substrate (5 mg) was used for the synthesis of these radiotracers. Raclopride is a dopamine D 2 /D 3 receptor antagonist and its carbon-11 labeled isotopologue, [ 11 C]raclopride ( [ 11 C]18 ), is commonly produced as a PET tracer in many PET radiochemistry facilities (Fig. 6a ) for evaluating the density or occupancy of the D 2 -dopamine receptor. Although the [ 11 C]ethyl iodide based N -ethylation method had been reported before for synthesizing this tracer at its early development stage [37] , the phenoxy group 11 C-methylation method using [ 11 C]CH 3 I/[ 11 C]CH 3 OTf as the radiosynthon has become the regular synthesis method for routine production of this clinically important tracer [38] , [39] , although the 11 C-carbonylation method was also intensively investigated [40] . In this research, FMDS 11 C-methylation approach was successfully implemented to synthesize this tracer. Using dual TBDMS attached precursor 17 , the 11 C-labeling and in situ deprotection of TBDMS group produced [ 11 C]raclopride, [ 11 C]18 , with 27.8 ± 2.2% yield after purification through the solid phase extraction (SPE) method, which is lower than reference reported methods [37] , [38] , [39] , [40] . Further optimizations in the future, such as changing TBDMS group to more labile TMS or TES groups and therefore decreasing 11 C-methylation reaction temperature, should help us to improve the production yield. Fig. 6: Practical synthesis of three radiotracers via FMDS 11 C-labeling approach. a [ 11 C]raclopride synthesis via 11 C-methylation of dual TBDMS attached precursor 17 ; b [ 11 C]succinic acid synthesis via 11 C-carboxylation of alkylsilane 6k and Al-Ni alloy reduction of intermediate [ 11 C ] 7 ; c [ 11 C]dichloroacetic acid synthesis via 11 C-carboxylation of alkylsilane 12g . Full size image Succinic acid is an endogenous dicarboxylic acid which had been identified as an oncometabolite [41] . Carbon-11 labeled succinic acid may have the potential to map the metabolic process of cancer cells and help cancer diagnosis, staging and re-staging [41] , [42] . Carbon-11 labeled dicarboxylic acids were synthesized by nucleophilic 11 C-cyanation and followed by basic hydrolysis [43] . However, this method requires an additional expensive and complex automated [ 11 C]HCN production module. In this study, the 4-ethoxy-4-oxobut-2-ynoic-[1- 11 C]acid, [ 11 C]7k , was first synthesized by FMDS 11 C-carboxylation method (described in Fig. 2 ). After two quick and efficient SPE purifications to remove unreacted [ 11 C]CO 2 , CsF and solvent, etc., the 11 C-intermediate, [ 11 C]7k , was eluted to the second reaction vial and mixed with Al-Ni alloy in basic solution for alkyne reduction (50 °C, 5 min) [44] . The desired [ 11 C]succinic acid, [ 11 C]19 , was obtained with a 50.1 ± 12.3% yield (Fig. 6b ) following acidification and filtration through a celite plug. Dichloroacetic acid (DCAA) is a small halogenated acetic acid analog, it can affect cancer cell metabolism and antagonize its growth by inhibiting mitochondrial pyruvate dehydrogenase kinases. DCAA has been investigated clinically for the treatment of various cancers (including brain, colon, breast, colorectal, and skin cancers). Its therapeutic applications and intriguing pharmacological properties have attracted a lot of attention from medical researchers [45] , [46] . The combination of PET imaging technique and 11 C-labeled DCAA, potentially, could facilitate researchers’ understanding of in vivo metabolic processes and pharmacokinetics of this low-price, low toxicity and promising cancer drug candidate. Employing FMDS 11 C-carboxylation protocol for synthesis of [ 11 C]13g (Fig. 4 ) followed by a quick SPE workup and semi-prep HPLC purification process, with only 5 min cyclotron beam time (producing 11.8 ± 4.2 GBq starting [ 11 C]CO 2 radioactivity), we obtained 1.1 GBq of the desired [ 11 C]DCAA, [ 11 C]13g , (RCY, 31.8 ± 3.1%) with over 99% radiochemical purity in a 35.7 ± 3.2 min synthesis process (Fig. 6c ). The product had A m of 71.7 ± 18.1 GBq/µmol (EOB), which should be satisfactory for oncological imaging studies in humans. The development of a robust FMDS 11 C-labeling strategy, although still in its early stages, opens up the potential for the synthesis of 11 C-labeled organic carboxylic acids and their derivatives directly using [ 11 C]CO 2 . The simplicity, high degree of reproducibility, and broad scope of the transformation of this approach, as showcased by the 11 C-labeling of various biologically interesting organic molecules, makes it a promising approach in radiotracer chemistry. In addition, the expansion of FMDS 11 C-labeling method using [ 11 C]CH 3 I as a radiosynthon is a beneficial supplement to current [ 11 C]CH 3 I/[ 11 C]CH 3 OTf based radiochemistry. The further extension and application of FMDS 11 C-labeling method to solve several long-standing problems in 11 C-radiotracer chemistry will be reported in due course. General procedures of [ 11 C]CO 2 production [ 11 C]CO 2 was generated by bombarding N 2 gas (360 psi 99.9999% pure N 2 doped with 0.5% O 2 ) via the 14 N (p,α) 11 C nuclear reaction using a EBCO TR-19/9 cyclotron. General bombardment conditions: 2–40 min beam time with 25 µA current (3.7–44.4 GBq; 100–1200 mCi). After the bombardment, target gas containing radioactivity was released and delivered to a home-made automated [ 11 C]CO 2 purification box for controlled trap and release of [ 11 C]CO 2 , where the [ 11 C]CO 2 was first trapped by a molecular sieve (MS) furnace at room temperature (200 mg molecular sieve 13X, 100/120 mesh, SUPELCO). Next, the furnace is heated to 190 °C and [ 11 C]CO 2 was released and delivered to the reaction vial using helium flow (10 mL/min). Once the radioactivity collected in the reaction vial plateaued, the delivery was stopped and [ 11 C]CO 2 production and collection was done. 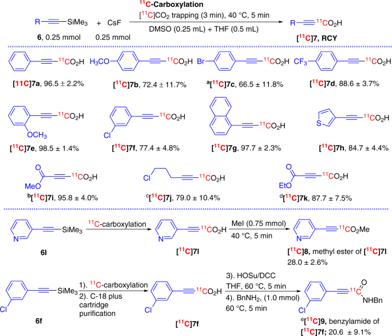Fig. 2: FMDS11C-carboxylation with sp-hybridized carbon attached trimethylsilanes. Unless otherwise indicated, the reported values are radiochemical yields (RCY,n= 3) of determined by radio-HPLC analysis of the crude product and the product identities were determined by co-injection with corresponding carbon-12 standards.aTHF (0.5 mL) + DMF (0.25 mL) were used;bReaction was maintained at r.t., 2 min;cDMSO was used as solvent;dPrecursor (0.029 mmol, 5 mg) and DMF (0.3 mL) were used for reactions. It took 3–4 min from end of bombardment (EOB) to end of the collection of [ 11 C]CO 2 in the reaction vial. General procedures of FMDS 11 C-carboxylation reaction Once the [ 11 C]CO 2 was ready, the [ 11 C]CO 2 delivery line with a 4-inch needle was inserted into a reaction vial containing the anhydrous fluoride reagent and solvent reaction mixture. The vial was equipped with outlet line (an ascarite trap was attached at the end for trapping escaped [ 11 C]CO 2 ). After confirmation of a stable helium flow (10 mL/min), the organosilane precursor was immediately added. The reaction vial was placed in a dose calibrator for measuring the collected radioactivity. Once the increase of radioactivity in the reaction vial plateaued, the [ 11 C]CO 2 delivery line and outlet line were removed immediately. The total activity trapped in the reaction vial was checked again, and recorded as starting radioactivity A 0 . When dimethylformamide (DMF), dimethylacetamide (DMA) and dimethyl sulfoxide (DMSO), as well as its mixture with tetrahydrofuran (THF) (1/1, v/v) were used as solvents for reactions, the trapping of radioactivity [ 11 C]CO 2 was generally efficient and the escaped [ 11 C]CO 2 collected by the ascarite trap at the outlet of the reaction vial was usually less than 10%. When only THF or THF/dichloromethane (DCM) (3/1, v/v) was used as the reaction solvent, a cooling bath was used (−70–0 °C) to keep reaction vial cool and escaped radioactivity was also minimal (< 10%). After maintaining the reaction mixture at the desired temperature with stirring for a specific time frame (normally 2–10 min), the reaction was quenched by addition of an acidic solution (1 mL, CH 3 CN/H 2 O/formic acid, 90/9/1; or 0.1 M HCl aqueous solution). The unreacted [ 11 C]CO 2 was purged from the reaction vial with a gentle stream of helium (2–5 psi) and trapped in a second ascarite trap. When the radioactivity collected in this ascarite trap became constant ( A leak ), the remaining radioactivity in the reaction vial was again measured and recorded as A left . After that, a small portion of solution was removed from reaction vial (0.1–0.2 mL) and diluted in a sample vial pre-loaded with an acidic solution (1 mL, CH 3 CN/1% formic acid, 90/10). Next, an analytical sample, which was a mixture of an aliquot of sample solution (usually 10 µL) and a product standard solution (usually 10 µL, 1 mg/mL solution), was injected into HPLC for analysis. The percentage of the radio-peak in the radio-chromatogram coincident with product reference UV peak was regarded as radiochemical purity (RCP). The radiochemical yield (RCY) was calculated by the equation [(RCP × A left )/ A 0 ] × 100%. The A 0 and A left were decay corrected values. If the reaction mixture was submitted for the purification process (solid phase extraction, anion/cation resins exchange method, semi-prep HPLC, or the combination of two of these methods), the total amount of radioactivity of purified product was recorded as A prod . The radiochemical yield (RCY, decay corrected) was calculated as ( A prod / A 0 ) × 100%. Total synthesis times were calculated from time point of finished collection of [ 11 C]CO 2 to the end of radiotracer purification process. [ 11 C]CH 3 I/[ 11 C]CH 3 OTf production [ 11 C]CO 2 was generated by bombarding N 2 gas (360 psi 99.9999% pure N 2 doped with 0.5% O 2 ) via the 14 N (p,α) 11 C nuclear reaction using a EBCO TR-19/9 cyclotron. General bombardment conditions for [ 11 C]CH 3 I/ [ 11 C]CH 3 OTf production: 5–40 min beam time with 25 µA current. After the bombardment, target gas containing radioactivity was released and delivered to a GE TRACERlab FXC automatic synthesizer to convert [ 11 C]CO 2 to [ 11 C]CH 3 I or [ 11 C]CH 3 OTf. It took 16–18 min from end of bombardment (EOB) to finish the collection of [ 11 C]CH 3 I or [ 11 C]CH 3 OTf radioactivity in the reaction vial. General procedures of FMDS 11 C-methylation reaction FMDS 11 C-methylation experimental process was the same as described for FMDS 11 C-carboxylation reactions except for that there was no unreacted [ 11 C]CO 2 exclusion process since unreacted [ 11 C]CH 3 I or by-product [ 11 C]CH 3 OH dissolved well in the reaction mixture and there was no leakage of radioactivity detected during the sampling process after the 11 C-methylation reaction. 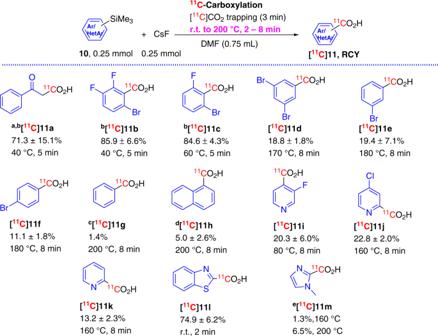Fig. 3: FMDS11C-carboxylation with sp2-hybridized carbon attached trimethylsilanes. aSolvent DMF (0.25 mL) + THF (0.5 mL), precursor is sp2-hybridized carbon attached silyl enol ether;bPrecursors are highly moisture sensitive;cThere was no detected product at 150 and 160 °C;dPrecursor 10 mg (0.05 mmol) in DMF (0.3 mL) (n= 4 for RCC);etert-Butyldimethylsilyl attached 1-methylimidazole was used as precursor; there was no product detected at 120 °C, 8 min for all reactions. When [ 11 C]CH 3 I or [ 11 C]CH 3 OTf was ready, the delivery line with a 4-inch needle was inserted into a reaction vial containing the anhydrous fluoride reagent and solvent reaction mixture equipped with outlet line. The organosilane precursor was immediately added. The reaction vial was placed in a dose calibrator for measuring the collected radioactivity. Once the increase of radioactivity in the reaction vial plateaued, the [ 11 C]CH 3 I or [ 11 C]CH 3 OTf delivery line and airflow outlet line were removed. The total activity trapped in the reaction vial was checked again as starting radioactivity A 0 . 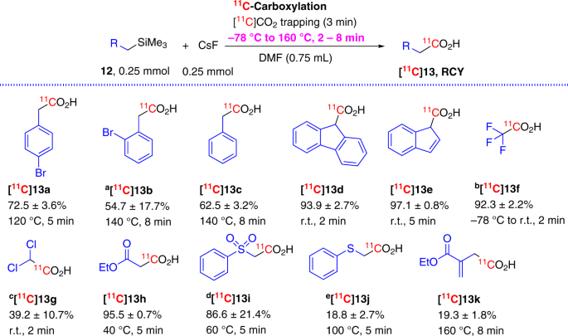Fig. 4: FMDS11C-carboxylation with sp3-hybridized carbon attached trimethylsilanes. aPrecursor (0.05 mmol, 12 mg), DMF (0.3 mL);bReaction vial was maintained at r.t. for 2 min after [11C]CO2collection was done at −78 °C, THF as solvent;cSolvent DMF (0.25 mL) + THF (0.5 mL);dPrecursor is highly moisture sensitive;eRCY based onn= 4. After keeping the reaction mixture stirring under desired temperature for a specific time (generally 2–10 min), the reaction mixture was measured again to have total radioactivity A 0 ′ (The value of A 0 ′ was supposed to equal as A 0 after decay correction since unreacted [ 11 C]CH 3 I or by-product [ 11 C]CH 3 OH dissolved well in the reaction mixture. However, it was found that the value of A 0 ′ was slightly less than the value of A 0 after decay correction in some experiments. It is most likely because of the small leakage of [ 11 C]CH 3 I or by-product [ 11 C]CH 3 OH from reaction vial.) A small portion of reaction mixture (~0.1 mL) was removed and diluted with an acidic solution (CH 3 CN/1% formic acid, 90/10) in a septa cap sealed glass vial; the radioactivity of this sample was counted and recorded. Next, an analytical sample, which was a mixture of an aliquot of sample solution (usually 10 µL) and a product standard solution (usually 10 µL, 1mg/mL solution), was analyzed by analytical HPLC. The percentage of radio-peak in radio-chromatogram coincident with the product reference UV peak was regarded as radiochemical purity (RCP) and also as radiochemical yield (RCY, decay corrected) if A 0 ′ = A 0 , or RCY = RCP × ( A 0 ′/A 0 ) at the case of A 0 ′ < A 0 . If the reaction mixture was submitted for the purification process (solid phase extraction, semi-prep HPLC, anion/cation resins exchange method, or the combination of two of these methods), the total amount of radioactivity of purified product was recorded as A prod . The radiochemical yield (RCY, decay corrected) was calculated as ( A prod / A 0 ) × 100%. Total synthesis times were calculated from EOB to the end of radioactive product collection after the purification. 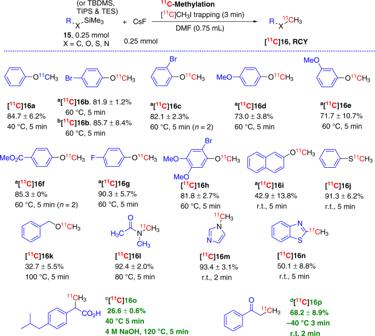Fig. 5: FMDS11C-methylation. atert-Butyldimethylsilyl (TBDMS) group attached compounds as labeling precursors;bTriisopropylsilyl (TIPS) group attached compound as labeling precursor.cTriethylsilyl (TES) group attached ethyl ester as labeling precursor; [11C]CH3I was collected at r.t., 3 min, then 40 °C, 2 min; Next saponification: 4 M NaOH, 120 °C, 5 min; products were purified by semi-prep HPLC.dTASF was used as fluoride source, THF (0.5 mL)/DCM (0.25 mL) was used as solvent, [11C]CH3I was collected at −40 °C, 3 min, reaction mixture was left at r.t., 2 min, products were purified by semi-prep HPLC; starting radioactivity of [11C]CH3I: 7.3 ± 2.67 GBq; total synthesis time: 37.7 ± 1.2 min; radiochemical purity (RCP) > 99% andAm: 29.7 ± 10.9 GBq/µmol (end of bombardment, EOB). 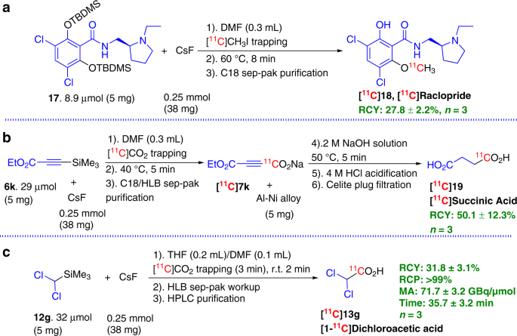Fig. 6: Practical synthesis of three radiotracers via FMDS11C-labeling approach. a[11C]raclopride synthesis via11C-methylation of dual TBDMS attached precursor17;b[11C]succinic acid synthesis via11C-carboxylation of alkylsilane6kand Al-Ni alloy reduction of intermediate [11C]7;c[11C]dichloroacetic acid synthesis via11C-carboxylation of alkylsilane12g. Molar activity ( A m ) A m values, decay corrected back to EOB and recorded in GBq/µmol, were determined from the carbon-11 activity in the HPLC product peak and the mass of compound.